Interaction-induced decay of a heteronuclear two-atom system Two-atom systems in small traps are of fundamental interest for understanding the role of interactions in degenerate cold gases and for the creation of quantum gates in quantum information processing with single-atom traps. One of the key quantities is the inelastic relaxation (decay) time when one of the atoms or both are in a higher hyperfine state. Here we measure this quantity in a heteronuclear system of 87 Rb and 85 Rb in a micro optical trap and demonstrate experimentally and theoretically the presence of both fast and slow relaxation processes, depending on the choice of the initial hyperfine states. This experimental method allows us to single out a particular relaxation process thus provides an extremely clean platform for collisional physics studies. Our results have also implications for engineering of quantum states via controlled collisions and creation of two-qubit quantum gates. The studies of two-atom systems in small traps attract a great deal of interest, in particular for engineering of quantum states via controlled collisions and creation of quantum gates in quantum information processing with a set of single-atom traps [1] , [2] . The crucial points are the decoherence time and the lifetime related to the interaction-induced inelastic decay of a higher hyperfine state. On the other hand, this type of inelastic processes, in particular heteronuclear ones, are important for the creation of multi-species quantum degenerate systems [3] , for obtaining ultracold heteronuclear molecules [4] , and for ultracold chemistry [5] . In homonuclear systems, the inelastic processes have been well studied from large ensembles of atoms to a few and even two atoms [6] , [7] , [8] . However, in the studies of inelastic heteronuclear collisions in a trapped gas [9] the main obstacle is the simultaneous presence of a large variety of loss mechanisms, which complicates the analysis. In magneto-optical traps where many heteronuclear systems have been studied [10] , [11] , [12] , [13] , [14] , [15] , [16] , aside from collisional processes one has radiative escape. In optical dipole traps there are homonuclear inelastic collisions [17] , [18] , [19] , and at sufficiently large densities, three-body recombination becomes important [20] . It is thus crucial to perform experiments allowing one to single out a particular inelastic process. This is done in the present paper. We study a two-atom system of different isotopes of rubidium (single 85 Rb and single 87 Rb) in a micro optical trap. One of them or both are in a higher hyperfine state, and we measure the corresponding rate of inelastic relaxation accompanied by the loss of the atoms. The homonuclear collisions are absent and our measurements give pure loss rates of specific hyperfine heteronuclear collisions. The experiments are done at temperatures close to the border of the ultracold limit (tens of microkelvins) and are supported by finite temperature coupled channel calculations. Our work can be easily extended to other alkali atoms, even to atom–molecule collisions [21] , [22] , thus allowing further understanding of heteronuclear collisions, a precise test of atomic collisional theory, and applications to quantum information processing. Experimental setup and results Our two-atom heteronuclear system is composed of a single 85 Rb and a single 87 Rb in a micro optical dipole trap (ODT), and there are three important points in the experiment. The first one is a sequential trapping of a single 87 Rb in a static ODT and a single 85 Rb in a movable ODT [23] , and we make sure that two atoms of different isotopes are actually trapped (see Fig. 1 and Methods). Second, we shift the movable ODT to overlap with the static one, and adiabatically turn off the movable trap. We get 87 Rb and 85 Rb in one trap with probability of about 95%. The third point is that the collisional blockade [24] does not allow us to detect the presence of 87 Rb or 85 Rb when both of them are in the same trap. Therefore, we first have to kick out one of the atoms to detect the presence of the other one. By optimizing this procedure we have minimized unwanted atom losses to <3%. 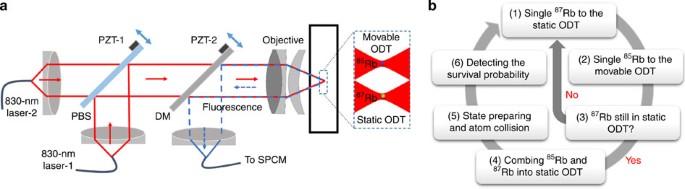Figure 1: Experimental setup and measurement time sequence. (a) Schematic diagram of the experimental setup. Two 830-nm lasers are collimated, combined by a polarizing beam splitter (PBS) and then strongly focused by an objective (Linos, HALO30) into the vacuum chamber to form two ODTs. The movable ODT is from 830-nm laser-1 and can be shifted to overlap with the static ODT (from 830-nm laser-2) by controlling piezoelectric ceramic transducer (PZT)-1. The fluorescence of trapped single atoms is collected by the same objective, separated from dipole lasers by a dichroic mirror (DM) and guided to single-photon-counting module (SPCM) for detection. PZT-2 controls the fluorescence-collecting region. A detailed description can be found in Methods. (b) Time sequence in the experiment. Each survival probability in our experiment is the result from 300 repeated measurements. Figure 1: Experimental setup and measurement time sequence. ( a ) Schematic diagram of the experimental setup. Two 830-nm lasers are collimated, combined by a polarizing beam splitter (PBS) and then strongly focused by an objective (Linos, HALO30) into the vacuum chamber to form two ODTs. The movable ODT is from 830-nm laser-1 and can be shifted to overlap with the static ODT (from 830-nm laser-2) by controlling piezoelectric ceramic transducer (PZT)-1. The fluorescence of trapped single atoms is collected by the same objective, separated from dipole lasers by a dichroic mirror (DM) and guided to single-photon-counting module (SPCM) for detection. PZT-2 controls the fluorescence-collecting region. A detailed description can be found in Methods. ( b ) Time sequence in the experiment. Each survival probability in our experiment is the result from 300 repeated measurements. Full size image Depending on the hyperfine states of 87 Rb and 85 Rb, there are three inelastic decay processes: We have not set a magnetic field, and for each atomic spin F in the initial state of the collision the states with all possible values of the spin projection M F are likely equally populated. The energy released in the inelastic processes A, B and C is about several GHz and it exceeds the trap depth U 0 by more than two orders of magnitude. Therefore, both atoms are ejected from the trap as a result of the inelastic relaxation. In most of our experiments the trap depth is U 0 =0.6 mK, which in our configuration provides the radial trap frequency ω ρ /(2 π )=38.8±0.1 kHz and the axial trap frequency ω z /(2 π )=3.2±0.1 kHz. We measure the survival probability P ( t ) for the atoms to remain in the trap at time t (see Fig. 2 ). For each t we execute 300 repetitions of the loop sequence of Fig. 1b . In the case of A and B processes the decay is strongly dominated by the interaction-induced spin relaxation. The probability P ( t ) is then described by an exponential time dependence. Within <10% of uncertainty the experimental data can be fitted with an exponential function P = w exp(− t / τ )+ w 0 . The presence of the offset w 0 has several reasons discussed in detail in Methods. First of all, the two-atom system is obtained with 95% probability, and there are traps with only one atom that remains trapped on a much longer timescale (about 11 s (ref. 25 )) than the collisional lifetime τ . Second, for the A and C processes doubly polarized pairs (for each atom the spin projection is equal to the spin) can decay only due to weak spin–spin or spin–orbit interactions that may change the spin projection of the pair, and the polarized pairs practically remain stable on the timescale of our experiment. For the B process, however, the doubly polarized pairs efficiently relax due to the channel leading to the formation of 87 Rb( F =1) and 85 Rb( F =3). 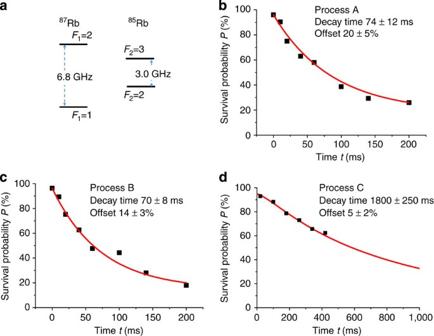Figure 2: Experimental data for the decay rates. (a) Energy levels of hyperfine states of87Rb and85Rb. (b–d) Survival probabilityPversus timetfor the A, B and C collisions, respectively. The measurements are done for the survival probability of87Rb after kicking out85Rb. The black squares are experimental data, with each point being the result from 300 repeated measurements. In (b,c) the solid curves show a fit by the formulaP=wexp(−t/τ)+w0, and the error in the decay time indicates the s.d. when using the fit ofP(t) by the exponential formula. In (d) the solid curve is a fit with the numerical solution of the rate equations including single-atom spin relaxation. The error in the decay time shows the uncertainty originating from the uncertainty in the single atom spin relaxation timeτrentering the rate equations (see Methods). The data are collected at the trap depthU0=0.6 mK and the initial temperaturesT87=35±3 μK,T85=15±1 μK. Figure 2: Experimental data for the decay rates. ( a ) Energy levels of hyperfine states of 87 Rb and 85 Rb. ( b – d ) Survival probability P versus time t for the A, B and C collisions, respectively. The measurements are done for the survival probability of 87 Rb after kicking out 85 Rb. The black squares are experimental data, with each point being the result from 300 repeated measurements. In ( b , c ) the solid curves show a fit by the formula P = w exp(− t / τ )+ w 0 , and the error in the decay time indicates the s.d. when using the fit of P ( t ) by the exponential formula. In ( d ) the solid curve is a fit with the numerical solution of the rate equations including single-atom spin relaxation. The error in the decay time shows the uncertainty originating from the uncertainty in the single atom spin relaxation time τ r entering the rate equations (see Methods). The data are collected at the trap depth U 0 =0.6 mK and the initial temperatures T 87 =35±3 μK, T 85 =15±1 μK. Full size image The process C is much slower than A and B, and our measurements for this process have been made on a timescale of about 500 ms. In this case the decay is significantly influenced by single-atom spin relaxation, and we have to take it into account in the rate equations for extracting τ from our measurements (see Methods). The measured τ has about 15% of statistical uncertainty that decreases with increasing the executed loop numbers. Aside from single-atom spin relaxation, the value of τ is influenced by single-atom loss events. The heating rate in the dipole trap is about 20 μK s −1 (ref. 26 ) and it increases the collisional volume, thus slightly increasing the decay time τ . We estimate the overall uncertainty in our values of τ as about 20%. We also test that the result for τ does not depend on whether we kick out 85 Rb or 87 Rb for measuring P ( t ). Comparing Fig. 2c with Fig. 3a it is easy to conclude that not only relaxation times are very close to each other (see also Table 1 ) but also the functions P ( t ). We then vary the temperature for the A collisional process to test the dependence of τ on the effective volume (density) of atoms in the trap. As expected, the time τ increases with temperature and one can see this from the comparison of the results in Figs 2b and 3b . 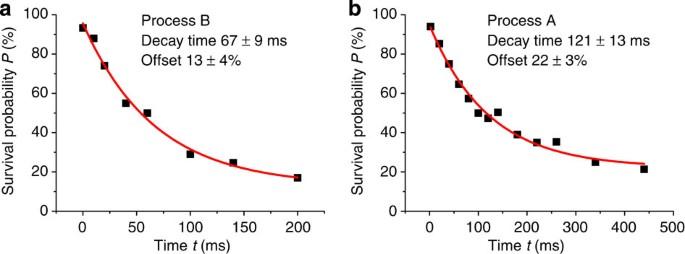Figure 3: The decay under different conditions. (a,b) Survival probabilityPversus timetfor the B and A collisions, respectively. The black squares are experimental data collected at the trap depthU0=0.6 mK, with each point being the result from 300 repeated measurements. The solid curves show a fit by the formulaP=wexp(−t/τ)+w0, and the error in the decay time indicates the s.d. when using the fit ofP(t) by the exponential formula. In (a) The measurements are done for the survival probability of85Rb after kicking out87Rb, and the initial temperatures areT87=35±3 μK andT85=15±1 μK. In (b)85Rb is kicked out, and the survival probability of87Rb is measured with the initial temperaturesT87=47±3 μK andT85=27±2 μK. Figure 3: The decay under different conditions. ( a , b ) Survival probability P versus time t for the B and A collisions, respectively. The black squares are experimental data collected at the trap depth U 0 =0.6 mK, with each point being the result from 300 repeated measurements. The solid curves show a fit by the formula P = w exp(− t / τ )+ w 0 , and the error in the decay time indicates the s.d. when using the fit of P ( t ) by the exponential formula. In ( a ) The measurements are done for the survival probability of 85 Rb after kicking out 87 Rb, and the initial temperatures are T 87 =35±3 μK and T 85 =15±1 μK. In ( b ) 85 Rb is kicked out, and the survival probability of 87 Rb is measured with the initial temperatures T 87 =47±3 μK and T 85 =27±2 μK. Full size image Table 1 Summary of the experimental and calculated results. The experiment is done with the trap depth U 0 =0.6 mK ( ω ρ /(2 π )=38.8 kHz, ω z /(2 π )=3.2 kHz). Full size table Theory and analysis The rate equations for the inelastic decay processes A, B and C can be written as where P ( t ) is the probability that at time t the atoms are still present in the trap, and τ is the relaxation (decay) time that we measure. These processes occur at interatomic distances of the order of or smaller than the radius of the interaction potential R e =( mC 6 / ħ 2 ) 1/4 ≈80 Å ( C 6 is the Van der Waals constant). At our trap frequencies and temperatures from 15 to 55 μK we have , and the motion of atoms in the trap is surely quasiclassical. In our trap configuration the extension of the wavefunction of the trapped atoms is the shortest in the radial direction , where m and ω ρ are the atom mass and radial trap frequency, respectively), and we still have the inequality Therefore, the decay (relaxation) time τ can be expressed through the relaxation rate constant α in free space: where is the effective volume, T eff = μ ( T 1 / m 1 + T 2 / m 2 ) is the effective temperature, with m 1 , m 2 and T 1 , T 2 being the masses and temperatures of 87 Rb and 85 Rb, respectively, and μ is the reduced mass. The rate constant α in equation (3) is averaged over the Boltzmann distribution of relative momenta k at effective temperature T eff : Note that due to elastic collisions between the atoms, the two-atom system eventually acquires an equilibrium temperature ( T 1 + T 2 )/2. However, it is different from the initial effective temperature T eff by <1%, and so will be the effective volume and the average value of α . At our temperatures, the quantity k T R e ∼ 0.5, where k T =( mT / ħ 2 ) 1/2 is the thermal momentum, so that we are close to the border of the s -wave-scattering limit. Therefore, in addition to the s -wave scattering, we took into account the scattering with higher orbital angular momenta. The rate constants α A , α B and α C for the processes A, B and C were calculated using the coupled channel method [4] , [27] at finite collision energies (see Methods). In the centre of mass reference frame, the Hamiltonian governing the collisions has the form where r is the interatomic distance, p is its conjugate momentum and ℓ is the orbital angular momentum operator. The interatomic interaction operator is given by V el ( r )= V s ( r ) P s + V t ( r ) P t , with P s and P t being projectors onto the electronic singlet and triplet states of the colliding pair of atoms. The term V hf = a 1 S 1 · I 1 + a 2 S 2 · I 2 is the hyperfine interaction, where S 1 , I 1 , a 1 and S 2 , I 2 , a 2 are the electron and nuclear spin operators and hyperfine constants for 87 Rb and 85 Rb, respectively. The total spin operators of the atoms are F 1 = S 1 + I 1 and F 2 = S 2 + I 2 , and the total spin operator of the pair is F = F 1 + F 2 . The Hamiltonian H of equation (6) conserves both the total spin F and its projection M F . It also conserves the orbital angular momentum ℓ and its projection M ℓ . The rate of inelastic spin relaxation occurring when at least one of the colliding atoms is in a higher hyperfine state can be expressed through the real and imaginary parts of the elastic scattering amplitude. The well-known formula for the inelastic rate constant [28] , averaged over the initial spin projections, is transformed to (see Methods): Accordingly, α A ≡ α (2, 3), α B ≡ α (2, 2), and α C ≡ α (1, 3). The quantity f ℓ ( F 1 , F 2 , F , k ) in equation (7) is the amplitude of elastic ℓ -wave scattering of these atoms at the total spin F . We apply the accumulated-phase method (see Methods) and calculate the accumulated-phase parameters from the known properties of homonuclear 87 Rb 87 Rb and 85 Rb 85 Rb collisions using mass scaling [27] . The main inaccuracy of our calculations stems from the choice of the accumulated phase, and we have checked that our results are stable within 5% when the value of this phase is varied by a few percent. The p -wave ( ℓ =1) contribution at our temperatures is comparable to the s -wave ( ℓ =0) one, but the contributions of the d -wave and higher partial waves are below 1%. Therefore, in the following we confine ourselves only to the s -wave and p -wave scattering. In Table 1 the results of the calculations for the processes A, B and C are compared with the experimental data. To show that finite temperature effects are important in our experiment we also present the rate constants calculated at T =0. For the fast A and B processes one sees an agreement between experiment and theory within the error bars of the experimental data. For the slow C process the calculated α is near the upper bound of the experimental value accounting only for statistical uncertainties. The reason for this small discrepancy is that the heating effect, although fairly small, still increases the effective volume so that the measured τ actually corresponds to slightly higher temperatures than the initial ones. This means that the experimental value of α at the initial temperatures should actually be slightly (by about 15%) higher than the one in Table 1 . The relaxation rates obtained in our work are rather high. In interesting experiments with spinor heteronuclear mixtures [29] , this places an upper limit of about n ∼ 10 12 cm −3 on the density if a higher hyperfine atomic state is involved. We should note, however, that the rate constant α C has a pronounced temperature dependence. At the temperatures used in this experiment, it is larger by about a factor of 4 than at T =0 (see Table 1 ). Our zero temperature result α C =0.8 × 10 −12 cm 3 s −1 is somewhat below the lower bound of the interval (1.2–4.5) × 10 −12 cm 3 s −1 found for the C process with 87 Rb( F 1 =1, M 1 =−1) and 85 Rb( F 2 =3, M 2 =3) in ref. 30 , which used old data for the interaction potentials. In experiments with ultracold clouds containing many atoms, the common temperature is ∼ 100 nK, which practically corresponds to T =0 limit in our calculations. We thus expect that an admixture of 85 Rb( F 2 =3) can be collisionally stable on a timescale of 100 ms in the gas of 87 Rb( F 1 =1) at densities approaching 10 13 cm −3 . Two-atom systems in small traps are convenient for the creation of heteronuclear molecules. In the gas mixture, Feshbach molecules of 87 Rb( F 1 =1, M 1 =−1) and 85 Rb( F 2 =2, M 2 =−2) have already been created [31] and they were undergoing losses due to collisional relaxation. In the two-atom system in a trap, the Feshbach molecule can be created by sweeping the magnetic field across the resonance like in experiments in an optical lattice [32] . For 87 Rb– 85 Rb, Feshbach resonances have been observed in the fields of hundreds of Gauss [31] and also predicted in the fields below 10 G ref. 33 . The rate of a spontaneous decay (dissociation) of a single Feshbach molecule in a trap due to spin relaxation [34] , [35] is proportional to α /〈 r 〉 3 , where α is the rate constant of relaxation in binary collisions and 〈 r 〉 is the size of the molecule [35] . With our relaxation rate constants α ∼ 10 −10 to 10 −12 cm 3 s −1 the decay time can be made on the level of tens of milliseconds, like in the case of 85 Rb– 85 Rb Feshbach molecules [35] . This is sufficient for using the two-photon-stimulated Raman adiabatic passage and transferring this molecule to the ground rovibrational state [36] . Our results may also have implications for engineering of quantum states and creation of two-qubit quantum gates based on controlled collisions in a system of single-atom traps [1] , [2] , [37] , in particular with respect to a proper selection of hyperfine atomic states. In our system, the relaxation time is τ = V eff / α and it strongly decreases with temperature, so that for atoms in the ground vibrational state τ may become of the order of the single-atom decoherence time τ dc . For collisional quantum gates the time τ dc and, hence, τ should be at least four orders of magnitude larger than the operational time τ op (ref. 38 ). The latter cannot be much smaller than the inverse interaction energy of the two atoms in the trap, and for atoms in the ground vibrational state one has τ op ∼ ħV eff / g , where g =4 πħ 2 a / m is the coupling constant for the elastic interaction, and a is the scattering length (this leads to τ op of about tens of microseconds at our trap frequencies, although for our present temperatures it is on the millisecond level). We thus have the condition: which immediately leads to the inequality For common values of g / ħ from 10 −9 to 10 −11 cm 3 s −1 equation (9) can be satisfied for doubly polarized atomic states, such as 87 Rb( F =2, M F =2) where g / ħ ∼ 10 −10 cm 3 s −1 , and the relaxation is caused only by weak spin–spin or spin–orbit interactions [32] leading to α <10 −14 cm 3 s −1 Another option would be to increase g by using a Feshbach resonance, although this can also increase inelastic losses. The advantage of our work is that we study collisions in a two-atom system, which allows us to single out a particular collisional process. In upcoming experiments we intend to trap single atoms with a farer detuned dipole laser (1,064 nm) to suppress the single-atom spin relaxation. We then prepare atomic states with given spin projections M F and cool the atoms down to the ground vibrational state [39] , [40] to execute the possibility of creating a quantum gate. Our work also paves a way to the creation of single heteronuclear molecules and to the studies of atom–molecule and molecule–molecule binary systems. Details of experimental methods In our experiment single atoms are trapped in micro ODTs that are formed by strongly focusing 830-nm lasers to a beam waist of about 2.1 μm. The dipole lasers follow the paths shown in Fig. 1a by the red solid lines. The movable ODT is initially 5 μm away and it can be shifted to overlap with the static ODT by changing the voltage of piezoelectric ceramic transducer-1. We detect trapped atoms by collecting the fluorescence in the trap region as shown by blue dashed lines. The fluorescence is coupled into a polarization-maintaining single-mode fibre (with the core diameter of 5 μm) for spatial filtering and is then guided to a single-photon-counting module (AQRH-14-FC). Owing to a moderate core diameter of the fibre and to a fairly large distance between the two traps, we can selectively collect the fluorescence from one of them. The disturbance from the other trap (crosstalk effect) is eliminated by properly adjusting the voltage of piezoelectric ceramic transducer-2. The experiment is executed following the time sequence shown in Fig. 1b . We first trap 87 Rb in the static ODT. During this step the movable ODT is off to prevent the loading of 87 Rb. Then we turn off the magneto-optical trap (MOT) of 87 Rb, and turn on the movable ODT and the 85 Rb MOT to execute step 2. The loading of a single 85 Rb may occur not only into the movable ODT but also into the static ODT, which leads to the loss of both 85 Rb and 87 Rb due to collisional blockade. Therefore, we do an extra check of the 87 Rb presence in the static trap in step 3. Only when 87 Rb is still trapped, we record the final result of the collision, otherwise we go back to step 1 and start loading again. To check that only 87 Rb is in the static trap and meanwhile only 85 Rb in the movable trap, we first detect the absence of the fluorescence of 87 Rb from the movable trap and the absence of fluorescence of 85 Rb from the static trap. This is followed by the fluorescence detection of 87 Rb and 85 Rb in the static and movable traps, respectively. In step 4 we first prepare 85 Rb in F 2 =2 and 87 Rb in F 1 =1 states to eliminate the unwanted collisional losses when switching off the MOT repumping lasers 1 ms before the MOT cooling lasers. For minimizing the heating effect we have optimized the process of transferring 85 Rb to the static trap. The transfer efficiency can go up to 98% and is limited by the detection efficiency and heating losses. The probability that 87 Rb survives when the movable trap approaches the static one and then is adiabatically switched off is also about 98%. The temperature is measured in this type of process by using the release and recapture technique [41] , [42] when one of the traps (either static or movable) is empty. In this way we create a heteronuclear two-atom system. After a certain time, we kick out one of the atoms from the trap using resonant lasers. Optimizing the laser intensities and shortening the pulse duration to 0.1 ms, we have minimized the unwanted losses to <3%. Eventually, we have succeeded in trapping two heteronuclear single atoms in the static ODT with about 95% probability. Analysis of the experimental data To confirm that the decay times τ A and τ B can be extracted by a simple exponential fit of the experiment data in Figs 2b,c and 3a,b , we numerically solved the rate equations taking into account single-atom spin relaxation. These are linear equations for the quantities representing the probabilities that both 87 Rb with spin F 1 and 85 Rb with spin F 2 are present in the trap at time t : We do not include single-atom loss in the rate equations, as the related loss time is about 11 s and it changes the simulated survival probability by <2% even at times t approaching 1,000 ms. For the time of single-atom spin relaxation we did an independent measurement, and the measured value is τ r =1,100±150 ms (see Fig. 4 ). 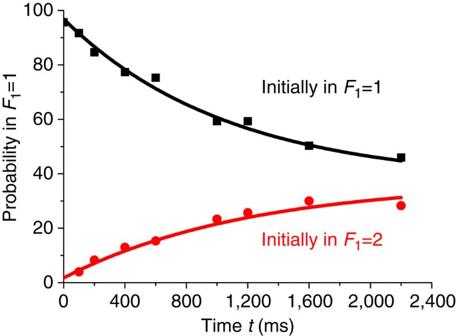Figure 4: Spin-relaxation measurement. We first prepare a single87Rb atom in the stateF1=1 (black squares) orF1=2 (red circles). After a timetwe kick out atoms that are populated in the stateF1=2 by using a resonant laser and then detect the survival probability of single atoms. Each data is averaged over 300 single atoms. The solid curves show a fit by the exponential formula: dP/dt∝exp(∓t/τr−t/τs), where the sign − is related to the black curve, the sign + to the red one, and the single-atom loss time isτs=11,000 ms. The fitted spin-relaxation time isτr=1,100±150 ms. Figure 4: Spin-relaxation measurement. We first prepare a single 87 Rb atom in the state F 1 =1 (black squares) or F 1 =2 (red circles). After a time t we kick out atoms that are populated in the state F 1 =2 by using a resonant laser and then detect the survival probability of single atoms. Each data is averaged over 300 single atoms. The solid curves show a fit by the exponential formula: d P /d t ∝ exp( ∓ t / τ r − t / τ s ), where the sign − is related to the black curve, the sign + to the red one, and the single-atom loss time is τ s =11,000 ms. The fitted spin-relaxation time is τ r =1,100±150 ms. Full size image The best fit with the experimental data for the process A in the conditions of Fig. 3b is obtained with τ A =129.5±1.5 ms at τ B =115±15 ms, τ C =1,800 ms and τ r =1,100 ms. The obtained τ A is consistent with the decay time of 121±13 ms given in Fig. 3b from the simple exponential fit. The simulations in the conditions of Figs 2b,c and 3a show that the best fitted τ A and τ B are larger than the exponential-fit decay times indicated in these figures by not more than 2 ms. The offsets of the fitted decay curves for the A and B processes in Figs 2 and 3 originate from several effects. They include the probability that there is only one atom in the trap ((5±2)%), the probability that 87 Rb( F 1 =2) undergoes a transition to the state with F 1 =1 due to Raman scattering of the dipole laser (about 5% for Figs 2b,c and 3a , and about 7% for Fig. 3b ), and for the A process the 6% probability that atom pairs are prepared in a doubly polarized state. All the offsets can be explained by these effects within our measurement uncertainty. For the slow process C the timescale is longer and the single-atom spin relaxation is more important, so that the time τ C can be extracted only from the best fit of the numerical solution of the rate equations with the experimental data. In Fig. 5 we display the results of the simulations in the conditions of Fig. 2d up to t =1,500 ms. The best numerical fit deviates from the experimental data by <10%. 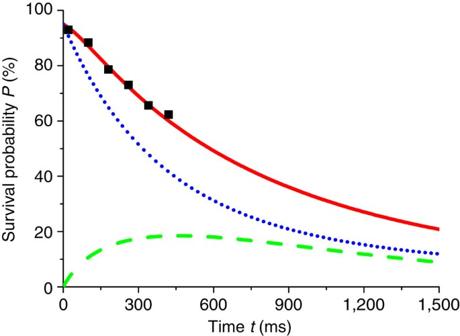Figure 5: Numerical fitting for the process C. We fit the experimental data (black squares) by numerical results from the rate equations for the process C. The red solid curve shows the survival probability of87Rb, the blue dotted curve shows the probabilityP13, and the green dashed curve is the probabilityP23+P22+P12. Figure 5: Numerical fitting for the process C. We fit the experimental data (black squares) by numerical results from the rate equations for the process C. The red solid curve shows the survival probability of 87 Rb, the blue dotted curve shows the probability P 13 , and the green dashed curve is the probability P 23 + P 22 + P 12 . Full size image Calculation of the inelastic rate constants At low temperature the inelastic spin relaxation occurs when at least one of the colliding atoms is in a higher hyperfine state. The rate constant of this process is given by [28] The quantity is the S -matrix element for the ℓ -wave scattering from the initial state i characterized by the atom spins F 1 , F 2 and their projections M 1 , M 2 to a final state f that has a lower internal (hyperfine) energy, so that there is an energy release in the inelastic scattering process. In equation (14) we also averaged over the initial spin projections M 1 and M 2 . Owing to the unitarity condition for the S -matrix elements we have: where S ii is the S -matrix element for elastic scattering in which the spin projections M 1 , M 2 remain the same, and S ii ′ is the S -matrix element for elastic scattering, which changes M 1 , M 2 to . Expressions for the S -matrix elements through the corresponding scattering amplitudes read [28] : The amplitudes are conveniently expressed through the amplitudes f ℓ ( F 1 , F 2 , F , k ) of elastic scattering of atoms with spins F 1 , F 2 at the total spin F of the pair: In the absence of a magnetic field the amplitudes f ℓ ( F 1 , F 2 , F , k ) do not depend on the total spin projection M . The Clebsch–Gordan coefficients, which appear in equation (17), satisfy the summation rule: Substituting equations (16) and (17) into equation (14), and making use of equation (18), we arrive at equation (7) of the main text: The amplitudes f ℓ ( F 1 , F 2 , F , k ) were calculated numerically using the coupled channel method [4] . Our implementation of this method is described in ref. 43 . The asymptotic behaviour of the scattering states is enforced at a distance of 1,000 a 0 , with a 0 being the Bohr radius. The accumulated-phase boundary condition is applied at r 0 =16 a 0 . It summarizes the short-range physics in the region of distances r < r 0 , where the triplet and singlet interaction potentials are poorly known, into six phase parameters. We calculate these parameters for heteronuclear 87 Rb 85 Rb collisions starting from the known data for homonuclear 87 Rb 87 Rb and 85 Rb 85 Rb collisions and using the mass scaling technique [27] , which exploits the fact that the Born–Oppenheimer electronic potentials V s and V t do not depend on the type of isotopes. The hyperfine coefficients a 1 and a 2 were taken from ref. 44 . Solving the coupled differential equations for the wavefunctions within the subspaces characterized by the conserved quantum numbers F , M we calculated all scattering amplitudes f ℓ ( F 1 , F 2 , F , k ) as functions of the incident relative momentum k . The calculated rate constants α ( F 1 , F 2 , k ) are then averaged over the thermal distribution of k according to equation (5). In Fig. 6 we present the calculated rate constants at temperatures from 0 to 100 μK and specify the s -wave, p -wave and d -wave contributions (the latter is below 1% at temperatures of our experiment, but at T =100 μK it is 4–5% for the A and B processes, and 10% for the C process). As one can see, the s -wave contribution slowly decreases with increasing temperature. However, the p -wave contribution significantly grows with T , which is expected. The role of the p -wave scattering is especially important for the C process, where it starts to dominate over the s -wave scattering already at T ∼ 15 μK. As a result, the total α C significantly increases with temperature. For the A and B processes the total α does not change much with increasing T as the decrease in the s -wave contribution is compensated by the p -wave contribution. 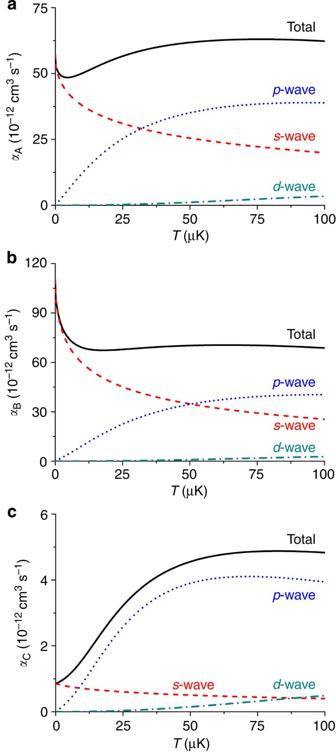Figure 6: Calculated rate constants. (a–c) The rate constantsαA,αBandαCare calculated at temperatures ranging from 0 to 100 μK, respectively. The black solid curves show the total rate constant, and the red dashed, blue dotted and dark cyan dash–dotted curves show thes-wave,p-wave andd-wave contributions, respectively. Figure 6: Calculated rate constants. ( a–c ) The rate constants α A , α B and α C are calculated at temperatures ranging from 0 to 100 μK, respectively. The black solid curves show the total rate constant, and the red dashed, blue dotted and dark cyan dash–dotted curves show the s -wave, p -wave and d -wave contributions, respectively. Full size image How to cite this article: Xu, P. et al. Interaction-induced decay of a heteronuclear two-atom system. Nat. Commun. 6:7803 doi: 10.1038/ncomms8803 (2015).